Atomically ordered solute segregation behaviour in an oxide grain boundary Grain boundary segregation is a critical issue in materials science because it determines the properties of individual grain boundaries and thus governs the macroscopic properties of materials. Recent progress in electron microscopy has greatly improved our understanding of grain boundary segregation phenomena down to atomistic dimensions, but solute segregation is still extremely challenging to experimentally identify at the atomic scale. Here, we report direct observations of atomic-scale yttrium solute segregation behaviours in an yttria-stabilized-zirconia grain boundary using atomic-resolution energy-dispersive X-ray spectroscopy analysis. We found that yttrium solute atoms preferentially segregate to specific atomic sites at the core of the grain boundary, forming a unique chemically-ordered structure across the grain boundary. Grain boundary (GB) segregation has been widely studied due to its importance in technological applications [1] , [2] , [3] , [4] , [5] , [6] , [7] , [8] , [9] , [10] , [11] . The enrichment of dopant atoms into GBs markedly affects the local structure, chemistry and thus governing overall properties of the materials [1] , [2] , [3] , [4] , [5] , [7] , [8] , [9] , [10] . Controlling GB segregation thus offers a promising strategy for materials engineering. To this end, an understanding towards the fundamental mechanisms of GB segregation is crucially important. Based on the Gibbs adsorption isotherm in thermodynamics, phenomenological understanding of GB segregation has been well established [12] . By further applying statistical mechanics with the consideration of site change energy between dopant and host atoms in the vicinity of the GB sites, the McLean model provided a general insight into GB segregation phenomena [12] . Although these theories give a general concept of GB segregation, atomistic mechanisms of how dopant atoms actually segregate to complex GB structures is still not fully clarified. This problem severely limits our ability to control GB segregation and resultant properties of many technologically important materials. Recently, it has become possible to directly visualize the ‘non-soluble’ impurity atoms segregated at GBs by using atomic-resolution scanning transmission electron microscopy (STEM) and spectroscopy [1] , [2] , [3] , [6] , [10] , [13] , [14] , [15] , [16] . The atomistic site-specific manner of impurity atom segregation has been proved for several ceramics, establishing a clear relationship between local GB non-solute segregation and resultant physical properties [1] , [3] , [10] . However, on the GB solute segregation, in which the dopant atoms can reside both at grain boundaries and within grain interiors, it has been extremely difficult to directly observe its structure and chemistry at atomic dimensions. At the same time, STEM–energy-dispersive X-ray spectroscopy (EDS) capabilities have steadily progressed. Ultrasensitive silicon drift detectors (SDDs) with much higher count rates allow the use of fine STEM probe, so that high quality, quantitative atomic-scale EDS mapping is now becoming possible [17] , [18] . This method may give us a chance to directly probe GB solute segregation phenomena by revealing preferred GB segregation sites of solute atoms. Here, we report an atomic-scale STEM–EDS mapping of a GB in yttria-stabilized zirconia (YSZ), which is one of the most important materials for electrolytes in solid oxide fuel cells [19] . In this study, a symmetric tilt GB with Σ3[110]/{111} orientation is selected as an initial attempt. It has been confirmed that Y atoms do segregate to this GB, but its structure is very coherent and simple [20] , which is ideal for TEM observations and theoretical calculations. Contrary to the previous models of continuous dopant solute segregation in GB, we show that Y segregation behaviour is atomic-site specific at the core of the GB. The detailed segregation process will be discussed in combination with results from large-scale Monte Carlo (MC) simulations. 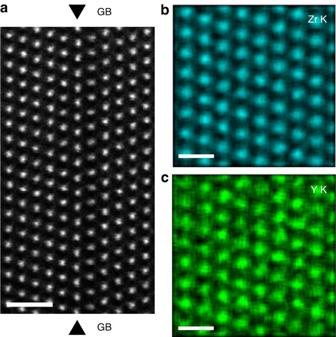Figure 1: Atomic structure of the grain boundary. (a) HAADF-STEM image of the GB. (b,c) Atomic resolution EDS elemental maps for (b) Zr K map, (c) Y K maps in the bulk region of the YSZ along [110] direction. Scale bar is 1 nm in (a) and 0.5 nm in (b,c). Characterization of site-dependent GB solute segregation Figure 1a shows a high angle annular dark-field (HAADF) STEM image of the Σ3[110]/{111} GB. The atomic column intensity in HAADF STEM image is approximately proportional to Z 2 ( Z represents the atomic number) [21] , so the bright contrast in the image represents the cation columns intermixed with Zr ( Z =40) and Y ( Z =39) atoms along this viewing direction. The GB atomic arrangement is in good agreement with the previous high-resolution TEM study [20] . However, it is impossible to distinguish Zr and Y atoms only from the HAADF STEM image. Figure 1: Atomic structure of the grain boundary. ( a ) HAADF-STEM image of the GB. ( b , c ) Atomic resolution EDS elemental maps for ( b ) Zr K map, ( c ) Y K maps in the bulk region of the YSZ along [110] direction. Scale bar is 1 nm in ( a ) and 0.5 nm in ( b , c ). Full size image To selectively observe Y atoms at the GB, a series of STEM–EDS mapping were performed. The low magnification STEM–EDS mapping revealed that Y atoms are homogeneously distributed inside the bulk regions, while they are enriched (Zr atoms decrease) at the GB vicinity (see Supplementary Fig. 1 ). Atomic-resolution STEM–EDS mapping on the bulk region is shown in Fig. 1b (Zr–K line) and Fig. 1c (Y–K line). The peak Y–K intensities are always found on the Zr atomic columns, and are almost uniform throughout the bulk region. This result indicates that the Y atoms homogeneously substitute the Zr atomic sites in the bulk regions. 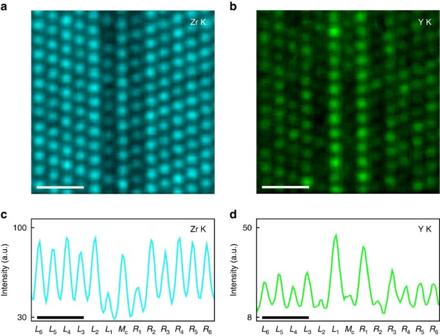Figure 2: Energy-dispersive X-ray spectroscopy maps and intensity profiles. (a,b) EDS elemental maps for (a) Zr K map and (b) Y K map. (c,d) Intensity profile (normalized by the total Zr and Y counts) by summing the X-ray counts in the maps in the direction parallel to the GB for (c) Zr K and (d) Y K. To show the subtle chemical variation more clearly, different scales are used for the two intensity profiles. Atomic layer number is listed in the bottom part of each figure. Scale bar is 1 nm. Figure 2a,b shows atomic-resolution STEM–EDS mappings around the GB core. Contrary to the bulk regions, the Y and Zr maps clearly reveal the formation of characteristic chemically ordered segregation structure. To better describe the segregation structure, we denote the cation planes as follows: cation mirror plane to be M c , the right-hand side of the M c plane to be R n planes and the left-hand side to be L n planes. Here, n is the sequential number as shown in the bottom of Fig. 2c,d . For the Y map, an apparent intensity increase can be found on the L 1 and R 1 planes, while for the Zr map, intensities decrease at these two planes. The intensity variation is more highlighted in the corresponding intensity profile normalized by the total Zr and Y counts, shown in Fig. 2c,d . These figures also visualize the subtle intensity variation across the GB. For the Y intensity line profile in Fig. 2d , slight increases in the L 3 , L 5 and R 3 planes were found, while clear decreases in the M C , L 2 and R 2 planes and slight intensity decreases in the L 4 and R 4 plane intensities were noted. On the other hand, for the Zr intensity line profile in Fig. 2c , an increase in the M C , L 2 , R 2 , L 4 and R 4 plane intensities can be recognized, while intensity decreases in the L 1 , R 1 , L 3 , R 3 and L 5 plane were evident. For the L 6 , R 5 and R 6 planes, both the Zr and Y intensities are almost constant, indicating the GB segregation structure extends as far as five or six layers adjacent to the M C plane. Note that the Y segregation is slightly stronger in the left-hand side of the M c plane. Figure 2: Energy-dispersive X-ray spectroscopy maps and intensity profiles. ( a , b ) EDS elemental maps for ( a ) Zr K map and ( b ) Y K map. ( c , d ) Intensity profile (normalized by the total Zr and Y counts) by summing the X-ray counts in the maps in the direction parallel to the GB for ( c ) Zr K and ( d ) Y K. To show the subtle chemical variation more clearly, different scales are used for the two intensity profiles. Atomic layer number is listed in the bottom part of each figure. Scale bar is 1 nm. Full size image The present atomic-resolution STEM–EDS mappings clearly reveal that Y segregation formed chemically ordered structure across the GB within the range of about 3 nm. Surprisingly, Y atoms are obviously depleted in some atomic column layers (that is, M c , L 2 and R 2 ). This indicates that Y atoms do not simply substitute all the cation sites around the GB. The unique site-dependent segregation pattern can be summarized as follows. Y atoms strongly segregate to the {111} atomic planes of L 1 and R 1 , and slightly to the L n and R n plane with odd number n . On the other hand, Y atoms are depleted in the M C plane and the L n and R n planes with even number n . Theoretical prediction of GB solute segregation behaviour In order to understand the observed characteristic segregation structure, systematic MC simulations combined with static lattice calculations were performed. 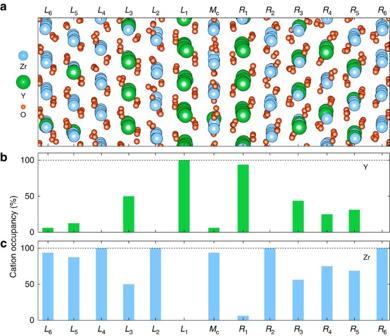Figure 3: Theoretical atomic structure at the grain boundary. (a) Atomic configuration of Y segregated GB predicted by theoretical calculations, along [110] direction. (b,c) atomic occupancy calculated from the predicted model structure for (b) Y atoms and (c) Zr atoms. Figure 3 shows the predicted equilibrium GB structure with Y segregation. The site occupancies of Zr and Y atoms across the GB are also shown in Fig. 3b,c , respectively. The chemically ordered segregation structure is well reproduced in the simulation. Zr atoms are almost fully substituted by Y atoms in the R 1 and L 1 planes and partially in the L 3 and R 3 planes. The chemical ordering almost disappears in the L 6 and R 6 planes. It is worth mentioning that, similar to the experimental result, the segregation level on the left-hand side of the GB is predicted to be slightly higher than the right-hand side. Figure 3: Theoretical atomic structure at the grain boundary. ( a ) Atomic configuration of Y segregated GB predicted by theoretical calculations, along [110] direction. ( b , c ) atomic occupancy calculated from the predicted model structure for ( b ) Y atoms and ( c ) Zr atoms. Full size image Based on the above simulation, we try to reveal the atomic-scale segregation processes. Here, GB atomic configurations are successively evaluated by the MC simulations varying Y concentrations from the lower to higher doping level (see Supplementary Fig. 2 and Supplementary Note 1 ). 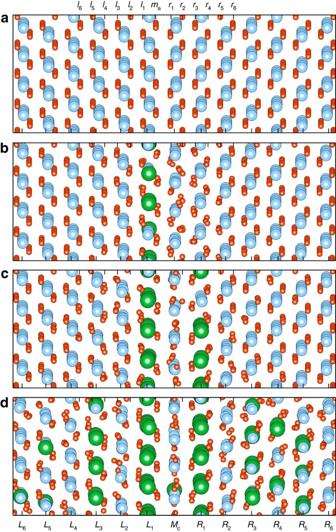Figure 4: Energetically favourable atomic arrangement. (a) The undoped model, (b) 6 Y, (c) 24 Y and (d) 60 Y atoms are introduced and O atoms are removed for maintaining charge neutrality. Figure 4 shows energetically favorable atomic configuration of the GB with different Y concentrations. Figure 4a shows the pristine model. It is seen that the plane distance between the M C and L 1 planes is slightly wider than other plane distances. This is because Zr sites in the L 1 plane are forced to have sevenfold coordination in this GB, while all other Zr sites are in eightfold coordination, resulting in the slight asymmetric GB structure [20] . At the initial stage of segregation modeled in Fig. 4b , Y ions preferentially occupy the L 1 plane. This ‘monolayer’ segregation structure can be related to the bond distortions at the L 1 plane sites due to the structurally formed sevenfold coordination sites. The occupation of Y ions at these sites effectively relieves total bond distortion and thus internal energy of the whole system. This way of site-dependent segregation is also reported in the previous studies of non-solute segregations [1] , [2] , [3] , [10] , [13] , [22] . Figure 4: Energetically favourable atomic arrangement. ( a ) The undoped model, ( b ) 6 Y, ( c ) 24 Y and ( d ) 60 Y atoms are introduced and O atoms are removed for maintaining charge neutrality. Full size image However, the present case involves more complicated factors for the segregation, namely the interactions between Y and O vacancies ( V O ), as discussed below. We labeled anion planes as m a , r n and l n (shown in the top of Fig. 4a ) following the same manner as in the cation planes, where the anion mirror plane m a is located in between M c and L 1 planes. As preferential Y segregation to the L 1 plane proceeds, V O segregate to the r 1 plane, which are located in the second-nearest neighbor sites relative to the Y ions in the L 1 plane. According to the previous studies, this geometric relationship between Y ions and V O is energetically favorable in the bulk of YSZ [23] , [24] . Therefore, the point defects interactions are likely to have significant effects on determining the preferred atomic arrangement at the GB. The accumulation of Y and V O causes larger oxygen bond distortion in the r 2 plane ( Fig. 4b ), which further accelerates segregation of both Y (on R 1 ) and V O (on r 2 ) in an ordered manner. V O preferentially segregates to the r 1 and r 2 planes, and consequently the two oxygen planes merged into form one oxygen plane ( Fig. 4c ). Then, the V O also start to segregate towards the bulk part of l 2 and r 5 sites at the same time, which further induces the V O segregation to the l 3 and r 6 sites and Y segregation to the L 3 and R 3 sites, forming the second-nearest neighbor pair Y– Vo configuration. In this way, Y atoms continue to segregate ( Fig. 4d ) and finally the GB reaches the unique segregation structures shown in Fig. 3 . Note that we have also experimentally confirmed the presence of V O in the GB by EDS (see Supplementary Fig. 3 ), which further support our conclusions. The present results provide atomic-scale insights into the GB solute segregation phenomena. Our study clearly reveals preferred segregation sites at the GB core even in the case of solute segregation. The interaction between Y and V O governs the subsequent segregation behaviour. The equilibrium segregation distribution is thus determined by these defect interactions coupled with GB geometries. It is worth mentioning that chemically ordered segregation structure is similar to a phase of Y 2 Zr 2 O 7 oxides with pyrochlore structure [25] , [26] . This indicates that solute segregation might induce a phase transition in the vicinity of GB. Previous studies suggest that extremely severe synthesis conditions such as high-pressure are indispensable for forming ordered Y 2 Zr 2 O 7 with the pyrochlore structure, but this structure has not been experimentally fabricated so far [25] . Therefore, we have provided a new possibility here: through artificial design of GB geometries and tailoring of GB segregation, new phases with novel properties may be created at GBs. Atomistic identification of subtle chemical difference at a GB, combined with theoretical calculations, shed light on the understanding towards solute segregation behaviours in GBs. It is demonstrated that GB solute segregation is driven by defect-GB interactions and the subsequent defect–defect interactions. These findings will be crucial for obtaining a complete picture of structure-property relationships at GBs in future. Furthermore, our results raise the possibility that segregation-induced GB phase transition is occurring, which might be a promising avenue to create novel phases inside materials that cannot be created by the current processing techniques. In addition, our approach may have broader utility in characterizing subtle chemical change at the atomic scale in materials science, solid-state physics and chemistry. Experimental procedure The YSZ bicrystal containing model GB was first fabricated by joining two YSZ (10 mol% Y 2 O 3 ) single crystals at 1,600 °C for 15 h in air, respectively [20] . TEM specimens were prepared by mechanical polishing and Ar-ion beam milling. The sample thickness is about 30 nm. The GB were observed using STEM (JEM-ARM200CF, JEOL Co. Ltd) operated at 200 keV. STEM–EDS mappings were acquired by scanning the beam near the GB, using the NSS3 software developed by the Thermo Fisher Scientific Inc. The STEM–EDS system is equipped with double SDD-EDS detectors and the solid angle for the whole collection system is about 1.7 sr. The probe size was 1.2 Å with the probe current of about 60 pA. Elemental maps were extracted with selected EDS energy for each element: Zr (using K α of 15.776 keV and K β of 17.668 keV) and Y (using K α of 14.958 keV and K β of 16.738 keV) were summed and the combined map is shown in the main text. The standard deviation of the integrated intensity profile are below ±2% of the total intensity in each sites. A typical EDS spectrum obtained is shown in the Supplementary Fig. 1 . In order to get high enough signals for the Zr and Y–K spectrum, the total acquisition time is about 48 min with the dwell time of 20 μs. The present results are reproducible and little affected by the experimental conditions used in this study (see Supplementary Figs 4 and 5 and Supplementary Note 2 ). Computational procedure A Σ3 [110]/{111} symmetric tilt GB model was constructed, which contains 512 Zr and 1024 O ions in the undoped model. The cell size is 96 × 14 × 13 Å and longest in the x -axis direction perpendicular to GB planes. The separation of 48 Å between the GB planes introduced by the periodic boundary condition is sufficient so that minimum-energy atomic configurations are unaffected by interactions between the GBs and point defects thereby. Y ions are substituted for Zr and charge compensating Vo are created for maintaining the charge neutrality. The dopant levels vary ranging from low to high dopant contents to pursue the process of point defect segregation. Total-energy calculations were carried out by static lattice methods implemented in the general utility lattice program (GULP) code [27] for all calculations. The Buckingham potential form with empirical parameters [26] was employed to evaluate short-range interactions. The parameters have been validated for various tilt GB models in previous studies [20] , [28] , [29] . The energy cutoff for short-range interactions was set to 15.0 Å for MC simulations and 20.0 Å for structural optimization. In order to obtain minimum-energy atomic configurations, we carried out site-interchange MC simulations with Metropolis algorithm [28] , [30] for cations (Y and Zr) and oxygen (O and Vo ), respectively at the same time, and subsequently all the ions were fully relaxed after each MC step. The favorable configurations were obtained varying dopant concentrations. The segregation energy and a comparison with the energetics obtained by the first-principles calculations can be found in the Supplementary Table 1 and Supplementary Note 3 . How to cite this article: Feng, B. et al . Atomically ordered solute segregation behaviour in an oxide grain boundary. Nat. Commun. 7:11079 doi: 10.1038/ncomms11079 (2016).